Developmental evidence for serial homology of the vertebrate jaw and gill arch skeleton Gegenbaur’s classical hypothesis of jaw–gill arch serial homology is widely cited, but remains unsupported by either palaeontological evidence (for example, a series of fossils reflecting the stepwise transformation of a gill arch into a jaw) or developmental genetic data (for example, shared molecular mechanisms underlying segment identity in the mandibular, hyoid and gill arch endoskeletons). Here we show that nested expression of Dlx genes—the ‘ Dlx code’ that specifies upper and lower jaw identity in mammals and teleosts—is a primitive feature of the mandibular, hyoid and gill arches of jawed vertebrates. Using fate-mapping techniques, we demonstrate that the principal dorsal and ventral endoskeletal segments of the jaw, hyoid and gill arches of the skate Leucoraja erinacea derive from molecularly equivalent mesenchymal domains of combinatorial Dlx gene expression. Our data suggest that vertebrate jaw, hyoid and gill arch cartilages are serially homologous, and were primitively patterned dorsoventrally by a common Dlx blueprint. The pharyngeal endoskeleton of jawed vertebrates (gnathostomes) was primitively segmented dorsoventrally into the palatoquadrate and Meckel’s cartilage in the mandibular arch, the hyomandibula and ceratohyal in the hyoid arch, and epibranchial and ceratobranchial elements in the gill arches. This ancestral (plesiomorphic) dorsoventral segmental organization is most readily observed, among extant gnathostomes, in the cartilaginous elasmobranch fishes (sharks, skates and rays) [1] , and differs considerably from the unjointed branchial basket and rostral velum of extant jawless vertebrates (cyclostomes, that is, lampreys and hagfishes) [2] . Gegenbaur’s classical hypothesis of jaw evolution by transformation of a rostral gill arch [3] was based on the apparent anatomical correspondence between the principal dorsal and ventral endoskeletal elements of the jaw, hyoid and gill arches of elasmobranchs, suggesting that these elements are serially homologous derivatives of a primitive branchial series. Framed in a modern phylogenetic context, the evolutionary origin of the jaw may be regarded as the culmination of stepwise anatomical changes to the rostral pharynx and nasohypophyseal complex along the gnathostome stem [2] , [4] , and comparative developmental studies of lampreys and gnathostomes have identified patterning disparities and morphogenetic constraints that account for differences in their oral apparatus [5] , [6] , [7] . Although this approach has yielded important insight into the developmental basis of morphological differences between mandibular arch derivatives in gnathostomes and cyclostomes, it remains difficult to polarize the sequence or direction of developmental patterning changes between these groups because there is no extant vertebrate outgroup for comparison. However, living representatives of both cartilaginous and bony fish lineages with plesiomorphic pharyngeal endoskeletal organization are available for study, and this renders testable the central tenet of Gegenbaur’s transformational hypothesis of jaw evolution—that the primitive endoskeletal elements of the upper and lower jaw, that is, the palatoquadrate and Meckel’s cartilage, are respectively serially homologous with the dorsal and ventral endoskeletal elements of the hyoid and gill arches. If these endoskeletal elements are indeed homologous, we would expect the molecular basis of their development to be shared across the mandibular, hyoid and gill arches, and we would further predict that such shared developmental mechanisms are more likely to be conserved in taxa with less divergent jaw, hyoid and gill arch endoskeletal morphology. In the mandibular and hyoid arches of both mouse [8] , [9] , [10] , [11] (a tetrapod, that is, a derivative of the sarcopterygian bony fish lineage) and zebrafish [12] (a teleost, that is, an actinopterygian bony fish), nested mesenchymal expression of the genes encoding the Dlx family of transcription factors (a ‘ Dlx code’) specifies dorsal versus ventral endoskeletal fate. In the mouse mandibular arch, Dlx1-2 are expressed throughout the entire arch, whereas Dlx3-6 are expressed only in the ventral half of the arch (with Dlx3-4 expression more ventrally restricted than Dlx5-6 expression [11] ). This nested Dlx expression, in turn, delineates domains of dorsal and ventral mesenchyme that form, among other structures, the derivatives of the palatoquadrate and Meckel’s cartilage (that is, the incus/ala temporalis and the malleus, respectively). For example, mice lacking Dlx1 and/or Dlx2 exhibit striking upper jaw malformations but effectively normal lower jaws [8] , [9] , whereas mice lacking both Dlx5 and Dlx6 exhibit a homeotic transformation of their lower jaw into an upper jaw [10] , [11] . There is currently little evidence from mouse or zebrafish that a Dlx code similarly patterns gill arch derivatives, though it is possible that such a patterning role has been modified or obscured with the evolution of their gill arch endoskeletal anatomy. In mouse, the ‘gill arches’ (that is, post-hyoid pharyngeal arches) no longer give rise to discrete epi- and ceratobranchial homologues, and the effects of Dlx gene loss-of-function on the morphology of gill arch endoskeletal derivatives are ambiguous [13] . In zebrafish, a full complement of gill arch endoskeletal derivatives does not form until after the endpoint of most molecular developmental studies [14] . Expression of Dlx orthologues has been reported in the gill arches of zebrafish [15] , [16] (and also in cichlids [17] , [18] , [19] ), though available data do not clearly demonstrate the existence of nested expression domains equivalent to those characterized in the zebrafish mandibular and hyoid arches [12] , and the role of Dlx genes in patterning the gill arch endoskeleton has not been assessed. To investigate putative primitive jaw and gill arch patterning mechanisms, we characterized expression of the Dlx gene family during pharyngeal arch development in three gnathostome taxa that have retained a relatively plesiomorphic pharyngeal endoskeletal organization: two cartilaginous (elasmobranch) fishes (the little skate, Leucoraja erinacea , and the small-spotted catshark, Scyliorhinus canicula ) and a basal actinopterygian bony fish (the Mississippi paddlefish, Polyodon spathula) . We show, in all three taxa, that an equivalent mesenchymal Dlx code is present in the mandibular, hyoid and gill arches. We also show that the principal dorsal and ventral segments of the jaw, hyoid and gill arch endoskeleton of the skate arise from equivalent dorsal and ventral domains of Dlx -coded mandibular, hyoid and gill arch mesenchyme. Overall, our data are consistent with the classical hypothesis of jaw–gill arch serial homology. Nested Dlx expression in elasmobranch pharyngeal arches We identified six Dlx genes each in skate and shark. Bayesian phylogenetic analysis of translated sequences ( Fig. 1 ) recovered six well-supported Dlx clades, each containing a single skate and shark Dlx orthologue. Consistent with previous findings in shark [20] , our analysis also recovered well-supported Dlx2/Dlx3/Dlx5 and Dlx1/Dlx4/Dlx6 clades, strongly supporting the 1:1 orthology of the six elasmobranch Dlx genes with the six mammalian Dlx genes. 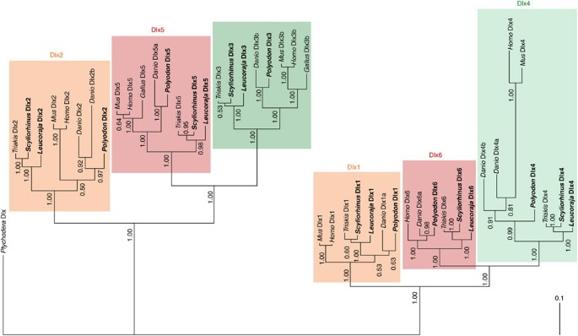Figure 1: Bayesian phylogenetic analysis of the gnathostome Dlx family. The skateLeucoraja erinacea, the sharkScyliorhinus caniculaand the paddlefishPolyodon spathulaeach possess six Dlx orthologues (in bold). Our analysis recovered six Dlx clades, each containing a single mouse (Mus), leopard shark (Triakis), skate (Leucoraja), dogfish (Scyliorhinus) and paddlefish (Polyodon) Dlx orthologue. All sequences (with the exception ofL. erinacea,S. caniculaandP. spathulasequences) were taken from the alignment of Stock20. A modified sequence alignment (including translatedL. erinacea,S. caniculaandP. spathulasequence fragments) was generated using the ClustalW algorhithm in MacVector, and phylogenetic analysis was performed using MrBayes 3.2. The analysis ran for 2,000,000 MCMC generations with a sampling frequency of 100. Numbers at the bases of clades are Bayesian posterior probabilities. Figure 1: Bayesian phylogenetic analysis of the gnathostome Dlx family. The skate Leucoraja erinacea , the shark Scyliorhinus canicula and the paddlefish Polyodon spathula each possess six Dlx orthologues (in bold). Our analysis recovered six Dlx clades, each containing a single mouse ( Mus ), leopard shark ( Triakis ), skate ( Leucoraja ), dogfish ( Scyliorhinus ) and paddlefish ( Polyodon ) Dlx orthologue. All sequences (with the exception of L. erinacea , S. canicula and P. spathula sequences) were taken from the alignment of Stock [20] . A modified sequence alignment (including translated L. erinacea , S. canicula and P. spathula sequence fragments) was generated using the ClustalW algorhithm in MacVector, and phylogenetic analysis was performed using MrBayes 3.2. The analysis ran for 2,000,000 MCMC generations with a sampling frequency of 100. Numbers at the bases of clades are Bayesian posterior probabilities. Full size image We next characterized Dlx gene expression in elasmobranch pharyngeal arches by whole-mount in situ hybridization from developmental stages 24–27. During these developmental stages in skate [21] and shark [22] , the pharyngeal arches are well formed (with four to six pharyngeal clefts perforated), the rostral-most pharyngeal cleft (spiracle) remains large and slit-like, and gill buds become apparent on all pharyngeal arches. Unlike in mouse and zebrafish, where nested Dlx expression has only been described in the mandibular and hyoid arches [8] , [9] , [10] , [11] , [12] , we observed nested Dlx expression in the developing mandibular, hyoid and gill arches in both skate ( Fig. 2a–g ; Supplementary Fig. S1 ) and shark ( Fig. 2h–n ; Supplementary Fig. S1 ). Dlx1 ( Fig. 2a ) and Dlx2 ( Fig. 2b ) are expressed throughout the entire dorsoventral extent of the mandibular, hyoid and gill arches (except a small intermediate domain of lower Dlx1 and Dlx2 expression in the middle of each arch in skate and shark, and very reduced Dlx1 expression in the ventral domain of each arch in shark). Expression of Dlx5 ( Fig. 2c ) and Dlx6 ( Fig. 2d ) is more ventrally restricted than that of Dlx1-2 , whereas expression of Dlx3 ( Fig. 2e ) and Dlx4 ( Fig. 2f ) is more ventrally restricted than that of Dlx5-6 . These expression patterns produce a combinatorial ‘ Dlx code’ in all pharyngeal arches ( Fig. 2g ), essentially indistinguishable from that characterized in the mammalian mandibular arch, that is, a dorsal domain of Dlx1 and Dlx2 expression, an intermediate domain of Dlx1, 2 , 5 and 6 expression and a ventral domain of Dlx1-6 expression. Sections reveal that Dlx expression is restricted to the neural crest-derived mesenchyme of the pharyngeal arches ( Fig. 2o–u ). Overall, these expression data indicate that nested, combinatorial expression of Dlx genes establishes molecularly equivalent dorsal, intermediate and ventral domains of mesenchyme in all pharyngeal arches (that is, in the mandibular, hyoid and gill arches) of elasmobranchs. 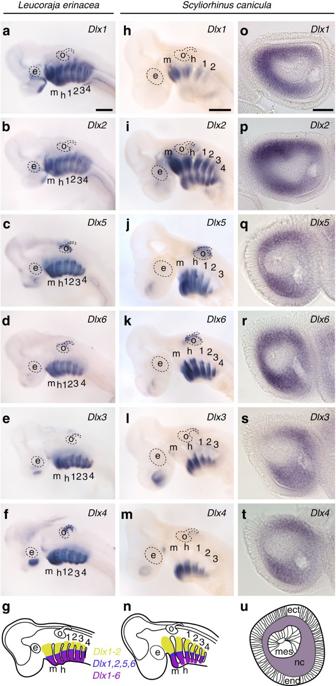Figure 2: NestedDlxexpression in the pharyngeal arches of elasmobranchs. (a–n) Whole-mountin situhybridization reveals that in the mandibular, hyoid and gill arches of the skateL. erinacea, (a,b)Dlx1-2, (c,d)Dlx5-6, and (e,f)Dlx3-4are expressed in progressively more ventrally restricted domains at stage 27, resulting in (g) nested, combinatorialDlxgene expression (that is, aDlxcode) in all pharyngeal arches. Similarly, nested expression of (h,i)Dlx1-2, (j,k)Dlx5-6and (l,m)Dlx3-4is observed in the mandibular, hyoid and gill arches of the sharkS. caniculaat stage 24, establishing (n) aDlxcode in all pharyngeal arches. (o–u) Vibratome sections afterin situhybridization reveal that pharyngeal arch expression ofDlx1-6is restricted to the neural crest-derived mesenchyme and excluded from ectoderm, endoderm and the mesodermal core. 1–4, gill arches 1–4; e, eye; ect, ectoderm; end, endoderm; h, hyoid arch; m, mandibular arch; mes, mesoderm; nc, neural crest-derived mesenchyme; o, otic vesicle; olf, olfactory organ. Scale bars, 500 μm (a–f); 500 μm (h–m); 25 μm (o–t). Figure 2: Nested Dlx expression in the pharyngeal arches of elasmobranchs. ( a – n ) Whole-mount in situ hybridization reveals that in the mandibular, hyoid and gill arches of the skate L. erinacea , ( a , b ) Dlx1-2 , ( c , d ) Dlx5-6 , and ( e , f ) Dlx3-4 are expressed in progressively more ventrally restricted domains at stage 27, resulting in ( g ) nested, combinatorial Dlx gene expression (that is, a Dlx code) in all pharyngeal arches. Similarly, nested expression of ( h , i ) Dlx1-2 , ( j , k ) Dlx5-6 and ( l , m ) Dlx3-4 is observed in the mandibular, hyoid and gill arches of the shark S. canicula at stage 24, establishing ( n ) a Dlx code in all pharyngeal arches. ( o – u ) Vibratome sections after in situ hybridization reveal that pharyngeal arch expression of Dlx1-6 is restricted to the neural crest-derived mesenchyme and excluded from ectoderm, endoderm and the mesodermal core. 1–4, gill arches 1–4; e, eye; ect, ectoderm; end, endoderm; h, hyoid arch; m, mandibular arch; mes, mesoderm; nc, neural crest-derived mesenchyme; o, otic vesicle; olf, olfactory organ. Scale bars, 500 μm ( a – f ); 500 μm ( h – m ); 25 μm ( o – t ). Full size image Nested Dlx expression in paddlefish pharyngeal arches To determine whether nested Dlx expression in elasmobranch gill arches is a derived feature of cartilaginous fishes, or a primitive gnathostome feature, we characterized Dlx gene expression in the pharyngeal arches of the paddlefish. Like elasmobranchs, paddlefishes have retained a relatively plesiomorphic pharyngeal arch organization. Expression analysis was carried out at developmental stage 34 (ref. 23 ). At this stage, the mandibular, hyoid and gill arches are well formed and externally recognizable, and the posterior expansion of the operculum (which derives from the hyoid arch) has not yet commenced. We identified six Dlx genes in paddlefish ( Fig. 1 ). As in skate and shark, we observed nested Dlx expression in the developing mandibular, hyoid and gill arches, with Dlx1 ( Fig. 3a ) and Dlx2 ( Fig. 3b ) expressed throughout the entire dorsoventral extent of the arches, Dlx5 ( Fig. 3c ) and Dlx6 ( Fig. 3d ) expressed in a more ventrally restricted pattern than Dlx1-2 , and Dlx3 ( Fig. 3e ) and Dlx4 ( Fig. 3f ) expression nested within the Dlx5 and Dlx6 domain. This combinatorial Dlx expression ( Fig. 3g ) is, again, reminiscent of the Dlx code of the mammalian mandibular arch. As in skate and shark, Dlx expression in all pharyngeal arches is restricted to the mesenchyme ( Fig. 3o–u ). Our expression data from elasmobranchs and paddlefish, therefore, indicate that the existence of molecularly distinct dorsal ( Dlx1-2 ), intermediate ( Dlx1, 2 , 5 and 6 ) and ventral ( Dlx1-6 ) domains of pharyngeal mesenchyme is not exclusively a developmental feature of the jaw and hyoid arch of bony fishes, but rather was a primitive feature of the mandibular, hyoid and gill arches in the last common ancestor of gnathostomes. 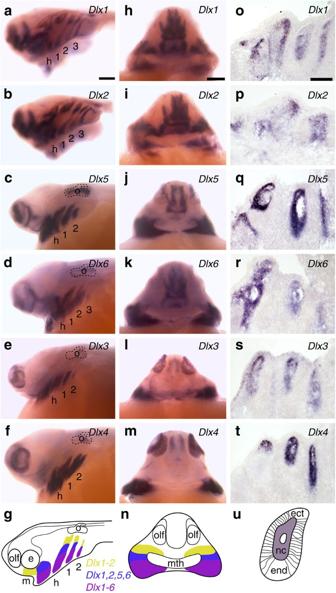Figure 3: NestedDlxexpression in the pharyngeal arches of paddlefish. Viewed laterally, whole-mountin situhybridization in stage 34P. spathulaembryos reveals expression of (a,b)Dlx1-2, (c,d)Dlx5-6and (e,f)Dlx3-4in progressively more ventrally restricted domains in the hyoid and gill arches, resulting in a nestedDlxcode in these arches, schematized ing. Frontal views of the same embryos reveal similarly nested expression patterns of (h,i)Dlx1-2, (j,k)Dlx5-6and (l,m)Dlx3-4in the mandibular arch, schematized inn. Sections reveal that paddlefish pharyngeal arch expression of (o–u)Dlx1-6is restricted to the neural crest-derived mesenchyme, and excluded from the ectoderm, endoderm and mesodermal core. 1–3, gill arches 1–3; e, eye; ect, ectoderm; end, endoderm; h, hyoid arch; m, mandibular arch; mes, mesoderm; mth, mouth; nc, neural crest-derived mesenchyme; o, otic vesicle; olf, olfactory organ. Scale bars, 200 μm (a–f); 200 μm (h–m); 50 μm (o–t). Figure 3: Nested Dlx expression in the pharyngeal arches of paddlefish. Viewed laterally, whole-mount in situ hybridization in stage 34 P. spathula embryos reveals expression of ( a , b ) Dlx1-2 , ( c , d ) Dlx5-6 and ( e , f ) Dlx3-4 in progressively more ventrally restricted domains in the hyoid and gill arches, resulting in a nested Dlx code in these arches, schematized in g . Frontal views of the same embryos reveal similarly nested expression patterns of ( h , i ) Dlx1-2 , ( j , k ) Dlx5-6 and ( l , m ) Dlx3-4 in the mandibular arch, schematized in n . Sections reveal that paddlefish pharyngeal arch expression of ( o – u ) Dlx1-6 is restricted to the neural crest-derived mesenchyme, and excluded from the ectoderm, endoderm and mesodermal core. 1–3, gill arches 1–3; e, eye; ect, ectoderm; end, endoderm; h, hyoid arch; m, mandibular arch; mes, mesoderm; mth, mouth; nc, neural crest-derived mesenchyme; o, otic vesicle; olf, olfactory organ. Scale bars, 200 μm ( a – f ); 200 μm ( h – m ); 50 μm ( o – t ). Full size image Skeletal fate of skate Dlx -expressing pharyngeal mesenchyme Nested Dlx expression in the pharyngeal arch mesenchyme of elasmobranchs and paddlefish is established before cartilage differentiation [24] , [25] . We therefore sought to determine if/how domains of Dlx -expressing mesenchyme correspond with endoskeletal anatomy in the mandibular, hyoid and gill arches. Using the lipophilic dye DiI, we labelled small populations of pharyngeal mesenchyme at three points along the dorsal–ventral axis of the mandibular, hyoid and first gill arch of stage 25–27 skate embryos: (1) within the dorsal Dlx1-2 -expressing domain; (2) within the ventral Dlx1-6 -expressing domain and (3) at the intermediate Dlx1-, 2 -, 5 - and 6 -expressing domain. We noted from our gene expression data that the intermediate domain corresponds with the point of maximum pharyngeal arch curvature in the mandibular, hyoid and first gill arch of L. erinacea ( Fig. 2g ). DiI injections targeting mesenchyme of the intermediate domain were therefore focused at the point of maximum arch curvature, whereas DiI injections targeting the dorsal and ventral domains were directed sufficiently dorsal or ventral to the point of curvature to ensure focal labelling of cells exclusively within the target domain. Embryos were cultured for up to 70 days and analysed histologically to assess the endoskeletal fates of each labelled mesenchymal cell population. After dorsal ( Dlx1-2 -expressing) mesenchyme was labelled ( Fig. 4a ), DiI-positive chondrocytes were located almost exclusively in the dorsal segments of each arch ( Fig. 4b ), for example, in the palatoquadrate within the mandibular arch ( Fig. 4c ), in the hyomandibula and pseudoepihyal within the hyoid arch ( Fig. 4e ), and in the epibranchial within the first gill arch ( Fig. 4g ). Conversely, after ventral ( Dlx1-6 -expressing) mesenchyme was labelled ( Fig. 4i ), DiI-positive chondrocytes were located almost exclusively in the ventral segments of each arch ( Fig. 4j ), for example, in Meckel’s cartilage within the mandibular arch ( Fig. 4k ), in the pseudoceratohyal within the hyoid arch ( Fig. 4m ) and in the ceratobranchial within the first gill arch ( Fig. 4o ). Finally, in embryos in which mesenchyme of the intermediate ( Dlx1-, 2 -, 5 - and 6 -expressing) domain was labelled ( Fig. 4q ), DiI-positive chondrocytes were found in both dorsal and ventral cartilages ( Fig. 4r ) in the mandibular ( Fig. 4s–u ), hyoid ( Fig. 4v ) and first gill arch ( Fig. 4x–z ). These findings indicate that pharyngeal endoskeletal segments classically regarded as serial homologues–for example, the dorsal palatoquadrate/hyomandibula+pseudoepihyal/epibranchials and the ventral Meckel’s cartilage/pseudoceratohyal/ceratobranchials–arise from equivalent domains of Dlx -expressing mesenchyme within their respective pharyngeal arches. 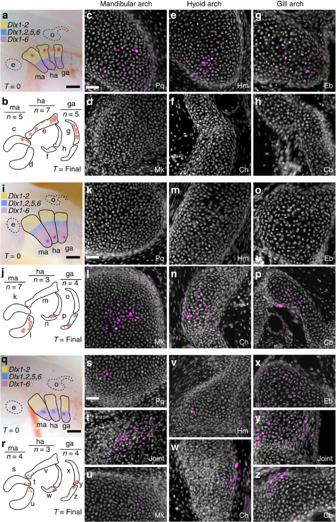Figure 4: Fate ofDlx-coded pharyngeal arch mesenchyme in skate. (a) Focal DiI labelling of the dorsal (Dlx1-2-expressing) mesenchyme of the mandibular, hyoid and first gill arch resulted in (b) regions of DiI-positive chondrocytes (red dots) concentrated in the dorsal segments of the jaw, hyoid and gill arch skeleton, for example, (c) in the palatoquadrate but (d) not in Meckel’s cartilage; (e) in the hyomandibula but (f) not in the pseudoceratohyal; and (g) in the epibranchial but (h) not in the ceratobranchial. Conversely, (i) focal DiI labelling of ventral (Dlx1-6-expressing) mesenchyme of the mandibular, hyoid and first gill arch resulted in (j) regions of DiI-positive chondrocytes (red dots) concentrated in the ventral segments of the jaw, hyoid and gill arch skeleton, for example, (k) not in the palatoquadrate, but (l) in Meckel’s cartilage; (m) not in the hyomandibula, but (n) in the pseudoceratohyal; and (o) not in the epibranchial, but (p) in the ceratobranchial. (q) Focal DiI labelling of intermediate (Dlx1-,2-,5- and6-expressing) mandibular, hyoid and gill arch mesenchyme resulted in (r) DiI-positive chondrocytes (red dots) concentrated at the point of articulation between the dorsal and ventral segments of the jaw, hyoid and gill arch skeleton, for example, (s–u) at the articulation between the palatoquadrate and Meckel’s cartilage; (v,w) in the hyomandibula and the pseudoceratohyal; and (x–z) at the articulation between the epibranchial and ceratobranchial. Dorsal and ventral skeletal elements of the mandibular, hyoid and first gill arch, therefore, arise from equivalent domains of combinatorialDlxexpression. All dorsal–ventral image pairs are from the same individual. Cb, ceratobranchial; Ch, pseudoceratohyal; e, eye; Eb, epibranchial; ga, gill arch; ha, hyoid arch; Hm, hyomandibula; ma, mandibular arch; Mk, Meckel’s cartilage; o, otic vesicle; Pq, palatoquadrate. Scale bars, 200 μm (a,i,q); 25 μm (c–h), (k–p), (s–z). Figure 4: Fate of Dlx -coded pharyngeal arch mesenchyme in skate. ( a ) Focal DiI labelling of the dorsal ( Dlx1-2 -expressing) mesenchyme of the mandibular, hyoid and first gill arch resulted in ( b ) regions of DiI-positive chondrocytes (red dots) concentrated in the dorsal segments of the jaw, hyoid and gill arch skeleton, for example, ( c ) in the palatoquadrate but ( d ) not in Meckel’s cartilage; ( e ) in the hyomandibula but ( f ) not in the pseudoceratohyal; and ( g ) in the epibranchial but ( h ) not in the ceratobranchial. Conversely, ( i ) focal DiI labelling of ventral ( Dlx1-6 -expressing) mesenchyme of the mandibular, hyoid and first gill arch resulted in ( j ) regions of DiI-positive chondrocytes (red dots) concentrated in the ventral segments of the jaw, hyoid and gill arch skeleton, for example, ( k ) not in the palatoquadrate, but ( l ) in Meckel’s cartilage; ( m ) not in the hyomandibula, but ( n ) in the pseudoceratohyal; and ( o ) not in the epibranchial, but ( p ) in the ceratobranchial. ( q ) Focal DiI labelling of intermediate ( Dlx1 -, 2 -, 5 - and 6 -expressing) mandibular, hyoid and gill arch mesenchyme resulted in ( r ) DiI-positive chondrocytes (red dots) concentrated at the point of articulation between the dorsal and ventral segments of the jaw, hyoid and gill arch skeleton, for example, ( s – u ) at the articulation between the palatoquadrate and Meckel’s cartilage; ( v , w ) in the hyomandibula and the pseudoceratohyal; and ( x – z ) at the articulation between the epibranchial and ceratobranchial. Dorsal and ventral skeletal elements of the mandibular, hyoid and first gill arch, therefore, arise from equivalent domains of combinatorial Dlx expression. All dorsal–ventral image pairs are from the same individual. Cb, ceratobranchial; Ch, pseudoceratohyal; e, eye; Eb, epibranchial; ga, gill arch; ha, hyoid arch; Hm, hyomandibula; ma, mandibular arch; Mk, Meckel’s cartilage; o, otic vesicle; Pq, palatoquadrate. Scale bars, 200 μm ( a , i , q ); 25 μm ( c – h ), ( k – p ), ( s – z ). Full size image A mandibular arch skeleton derived from Hox -negative neural crest mesenchyme is a shared, primitive feature of vertebrates [26] , [27] , but segmentation of the mandibular, hyoid and gill arch endoskeleton is observed only in gnathostomes. This must reflect the superimposition of a dorsoventral segmental patterning mechanism onto a pre-existing anteroposterior (that is, Hox -encoded) molecular identity in the pharyngeal arches of gnathostomes. We have demonstrated that an identical, nested pattern of Dlx gene expression (that is, a Dlx code) is present in the mandibular, hyoid and gill arches of elasmobranchs (shark, skate) and a basal actinopterygian bony fish (paddlefish). Furthermore, the principal dorsal and ventral endoskeletal segments of the mandibular, hyoid and gill arches of skate are derived from equivalent domains of this code. Given these findings, we suggest that the ancestral gnathostome jaw, hyoid and gill arch endoskeletal elements may indeed be classified as serial homologues, that is, the palatoquadrate and Meckel’s cartilage may be regarded as ‘epi’ (dorsal) and ‘cerato’ (ventral) components of the first pharyngeal arch ( Fig. 5 ). While shared patterns of gene expression do not necessarily provide evidence for the homology of associated anatomical structures [28] , [29] , we argue that the experimental demonstration in an elasmobranch of shared origins of the principal dorsal and ventral endoskeletal segments of the jaw, hyoid and gill arches from cell populations that co-express multiple developmental genes in identical patterns provides sufficient grounds for classifying these structures as serial homologues–that is, iterative features within an individual that correspond owing to a shared underlying gene regulatory network [30] , [31] , [32] , [33] . The demonstration of conservation of the Dlx code in the mandibular, hyoid and gill arches in representatives of both gnathostome lineages (that is, cartilaginous and bony fishes) further indicates that the iterative deployment of this patterning mechanism is a synapomorphy of jawed vertebrates. 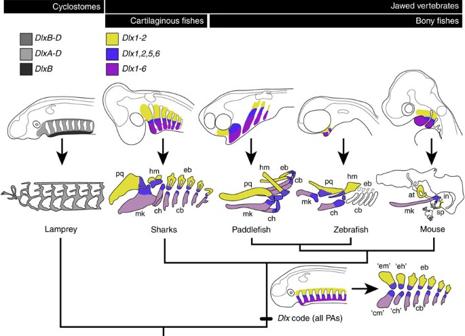Figure 5: Evolution of theDlxcode and serial homology of gnathostome pharyngeal endoskeletal elements. TheDlxcode arose along the gnathostome stem, and was primitively deployed in all pharyngeal arches. The evolutionary relationship between theDlxcode of gnathostomes and the nested expression ofDlxA-Din the pharyngeal arches of lamprey37remains unclear. Dorsal (Dlx1-2-expressing) and ventral (Dlx1-6-expressing) domains of theDlxcode would have primitively given rise to dorsal ‘epimandibular’, ‘epihyal’ and ‘epibranchial’ elements and ventral ‘ceratomandibular’, ‘ceratohyal’ and ‘ceratobranchial’ elements (in the mandibular, hyoid and gill arches, respectively), while intermediate (Dlx1-, 2-, 5- and6-expressing) domains would have given rise to the region of articulation between these elements. The primitive role for theDlxcode in patterning the mandibular, hyoid and gill arch endoskeletal segments has been conserved in elasmobranchs, and presumably in non-teleost actinopterygians (for example, paddlefish), while post-hyoid arch expression of theDlxcode has been modified or obscured in amniotes (for example, mouse) and possibly in teleosts. at, ala temporalis; cb, ceratobranchials; ‘ch’, hypothetical ceratohyal; ch, ceratohyal; ‘cm’, hypothetical ceratomandibula; eb, epibranchials; ‘eh’, hypothetical epihyal; ‘em’, hypothetical epimandibula; hm, hyomandibula; in, incus; mk, Meckel’s cartilage; pq, palatoquadrate; sp, styloid process; st, stapes. Figure 5: Evolution of the Dlx code and serial homology of gnathostome pharyngeal endoskeletal elements. The Dlx code arose along the gnathostome stem, and was primitively deployed in all pharyngeal arches. The evolutionary relationship between the Dlx code of gnathostomes and the nested expression of DlxA-D in the pharyngeal arches of lamprey [37] remains unclear. Dorsal ( Dlx1-2 -expressing) and ventral ( Dlx1-6 -expressing) domains of the Dlx code would have primitively given rise to dorsal ‘epimandibular’, ‘epihyal’ and ‘epibranchial’ elements and ventral ‘ceratomandibular’, ‘ceratohyal’ and ‘ceratobranchial’ elements (in the mandibular, hyoid and gill arches, respectively), while intermediate ( Dlx1-, 2-, 5 - and 6 -expressing) domains would have given rise to the region of articulation between these elements. The primitive role for the Dlx code in patterning the mandibular, hyoid and gill arch endoskeletal segments has been conserved in elasmobranchs, and presumably in non-teleost actinopterygians (for example, paddlefish), while post-hyoid arch expression of the Dlx code has been modified or obscured in amniotes (for example, mouse) and possibly in teleosts. at, ala temporalis; cb, ceratobranchials; ‘ch’, hypothetical ceratohyal; ch, ceratohyal; ‘cm’, hypothetical ceratomandibula; eb, epibranchials; ‘eh’, hypothetical epihyal; ‘em’, hypothetical epimandibula; hm, hyomandibula; in, incus; mk, Meckel’s cartilage; pq, palatoquadrate; sp, styloid process; st, stapes. Full size image Molecular developmental studies in lamprey have previously reported uniform (non-nested) expression of Dlx genes in all pharyngeal arches [34] , [35] , [36] . However, a recent study [37] describes nested expression of Hand (see also ref. 36 ), MsxB and four Dlx genes ( DlxA-D ) in the pharyngeal arches of lamprey, indicating a previously unrecognized dorsoventral patterning role for these factors in the pharyngeal arches of cyclostomes. While these findings demonstrate that the last common ancestor of vertebrates possessed pharyngeal arches with some degree of dorsoventral polarity [38] , it is likely that both cyclostomes and gnathostomes employ a combination of plesiomorphic and apomorphic developmental mechanisms in patterning their pharyngeal arches along the dorsoventral axis. For example, pharyngeal arch expression patterns of Hand and MsxB in lamprey are similar to those of orthologous genes during gnathostome pharyngeal arch development [39] , [40] , indicating that the role of these transcription factors in pharyngeal arch patterning is most likely conserved in cyclostomes and gnathostomes. However, discrepancy in the number of Dlx orthologues expressed in domains along the dorsoventral axis of the pharyngeal arches of lampreys and gnathostomes, and the unresolved orthology of lamprey and gnathostome Dlx genes [41] , precludes direct quantitative or qualitative comparisons of the lamprey pharyngeal ‘ Dlx prepattern’ with the gnathostome Dlx code. Thus, although differential expression of Dlx genes along the dorsoventral axis of lamprey pharyngeal arches may correspond with morphological/histological differentiation of the branchial basket [37] , [38] , the precise nature of the evolutionary relationship between the Dlx prepattern of lampreys and the Dlx code of gnathostomes remains unclear. Given the apparent correspondence of the dorsal and ventral domains of the Dlx code with the principal dorsal and ventral endoskeletal segments of each pharyngeal arch of elasmobranchs, the conservation of the Dlx code in the mandibular, hyoid and gill arches of paddlefish, and the above-mentioned differences between the expression/orthology of Dlx genes in lampreys and gnathostomes, we envision a scenario in which the Dlx code was initially established along the gnathostome stem, in all pharyngeal arches, likely coincident with the origin of pharyngeal endoskeletal segmentation ( Fig. 5 ). This would have established a primitive series of dorsal (‘epi’) and ventral (‘cerato’) skeletal elements—all patterned by a common Dlx blueprint—which would ultimately be modified to give rise to the jaw, hyoid and gill arch skeletal elements of the gnathostome crown group. The conservation of the Dlx code in the pharyngeal arches of elasmobranch fishes provides a molecular mechanism for the pronounced iterative pharyngeal endoskeletal segmentation that was the basis of Gegenbaur’s iconic hypothesis of jaw–gill arch serial homology over a century ago. Note added in proof: While our manuscript was in the proof stages, nested expression of Dlx genes in the pharyngeal arches of another shark species, Scyliorhinus torazame, was reported in a review by Takechi et al ., 2013, Semin. Cell Dev. Biol. http://dx.doi.org/10.1016/j.semcdb.2012.12.010 Embryo collection L. erinacea and S. canicula eggs were obtained from the Marine Biological Laboratory (Woods Hole, MA, USA) and the Station Biologique (Roscoff, France), respectively. Eggs were maintained in a flow-through seawater system at ambient temperature until stages 24–27 ( [21] , [22] ). P. spathula embryos were purchased from Osage Catfisheries (Osage Beach, MO, USA). Embryos were raised at ~22 °C in tanks with filtered and recirculating water (pH 7.2±0.7, salinity of 1.0±0.2 ppt) to stage 34 (ref. 23 ). All embryos were fixed in 4% paraformaldehyde for 4 h at room temperature or overnight at 4 °C, rinsed in PBS, dehydrated stepwise into 100% methanol or ethanol and stored at −20 °C. DiI labelling and histology DiI labelling in L. erinacea embryos was performed as described [42] . Embryos were fixed as described above, rinsed in PBS and stored at 4 °C in PBS with 0.02% sodium azide before embedding in paraffin wax and sectioning as described [43] . Sections were counterstained with DAPI (1 ng ml −1 for 10 min) before imaging. In situ hybridization, sectioning Whole-mount in situ hybridization in S. canicula ( Dlx1-6 , JX270824-29), L. erinacea ( Dlx1-6 , GenBank JX270812-17) and P. spathula ( Dlx1-6 , GenBank JX270818-23) was carried out as described [43] , [44] . Following in situ hybridization, L. erinacea and S. canicula embryos were cleared in 75% glycerol in PBS and embedded in 15% gelatin in PBS. Gelatin blocks were post-fixed in 2% paraformaldehyde overnight at 4 °C and sectioned at 40 μm using a Leica VT1000S vibratome. P. spathula embryos were incubated in 5% sucrose in PBS for 5 h at room temperature, then in 15% sucrose in PBS overnight at 4 °C, followed by an overnight incubation in pre-warmed 7.5% gelatin in 15% sucrose at 37 °C. Embryos were oriented in embedding moulds, which were immersed in a dry ice and isopentane solution for 1 min to freeze the gelatin, followed by cryosectioning at 20 μm. How to cite this article: Gillis, J. A. et al . Developmental evidence for serial homology of the vertebrate jaw and gill arch skeleton. Nat. Commun. 4:1436 doi: 10.1038/ncomms2429 (2013).